Silicate deposition during decomposition of cyanobacteria may promote export of picophytoplankton to the deep ocean Marine particles transport organic matter through the water column to the sediment where the organic matter can be buried. This pathway is one of the few natural removal mechanisms of CO 2 from the atmosphere over geological time. Picophytoplankton, major primary producers in the ocean, have until recently been thought unimportant regarding particle transport. Here we provide evidence that silicate is deposited on extracellular polymeric substance (EPS) associated with decomposing picophytoplankton. We also find that Si is enriched in a previously unexplored group of marine particles (called micro-blebs) from the deep-water column. The surprising similarity in morphology and composition between EPS-Si and micro-blebs suggests that EPS-Si may be a precursor of micro-blebs observed in the deep ocean. This previously unexplored source of silicon may be important to silicon cycling and may further enhance export of picophytoplankton to the deep ocean. Photosynthetic picophytoplankton (organisms 0.2–2 μm in size) are major primary producers that contribute more than 50% of the autotrophic biomass in oligotrophic ocean areas [1] , [2] . However, as a result of their small size, these picoplankton have long been considered to be less important to the transport of carbon from the atmosphere into the ocean that results from particle export [3] . Because of the widely observed quantitative relationship between particulate organic carbon (POC) and ballast minerals (for example, opal, carbonates and dust), biominerals from plankton like diatoms and coccolithophores are thought to contribute more, owing to density-driven particle sedimentation [4] , [5] . However, recent studies in oligotrophic areas have suggested that picophytoplankton are also important in transporting organic matter to the deep ocean [6] , [7] , [8] . The export mechanism is not clear, but it has been suggested that aggregation of picophytoplankton, and fecal pellets from grazers, can facilitate the settling of this material into the deep ocean [6] , [8] . To better understand mechanisms of cyanobacterial export in the marine environment, we conducted incubations of decomposing Synechococcus cells, during which we discovered that silicon can deposit on the detrital organic matter. This finding suggests a novel mechanism to explain our discovery of a new group of marine particles enriched in Si (micro-blebs) collected from a Bermuda Rise site in the North Atlantic Ocean. Degradation incubation of cyanobacteria In the incubations, we used two strains of the cyanobacterium, Synechococcus sp . (CCMP2370 and CCMP1334). These are open-ocean strains that were originally isolated from the Sargasso Sea where cyanobacteria are major primary producers for most of the year [2] . Cyanobacterial cells harvested during the late exponential phase were added to coastal seawater (Stony Brook Harbor, NY, USA) and allowed to decompose in the dark in the presence of natural microbial communities. Before adding cyanobacteria to the coastal seawater, mesozooplankton and larger zooplankton were removed by filtration so that microbial degradation dominated the incubations. Controls were also run where no cyanobacteria were added, and where the medium was sterilized before adding cyanobacteria. The seawater used in the incubations initially contained 1.8±1.4 μmol l −1 biogenic silicate (BSi) and 30±1.5 μmol l −1 dissolved silicic acid (H 4 SiO 4 ) ( Fig. 1 and Supplementary Fig. 1 ). Subsamples were collected over time to track microbial degradation of Synechococcus cells. 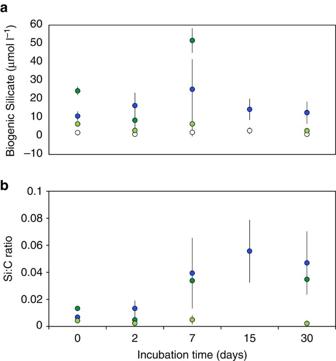Figure 1: BSi concentration and BSi/POC ratios. Changes in BSi concentration (a) and ratio of BSi to particulate organic carbon (b) during incubation ofSynechococcusCCMP2370 (dark green circles) and CCMP1334 (blue circles) in coastal seawater. CCMP2370 cells were incubated in autoclaved seawater (light green circles) in parallel to show any changes occurring in the absence of microbes. Coastal seawater (open circles) without addition ofSynechococcuscells was also incubated in parallel to show any changes occurring in natural seawater. The error bars represent standard deviation. Figure 1: BSi concentration and BSi/POC ratios. Changes in BSi concentration ( a ) and ratio of BSi to particulate organic carbon ( b ) during incubation of Synechococcus CCMP2370 (dark green circles) and CCMP1334 (blue circles) in coastal seawater. CCMP2370 cells were incubated in autoclaved seawater (light green circles) in parallel to show any changes occurring in the absence of microbes. Coastal seawater (open circles) without addition of Synechococcus cells was also incubated in parallel to show any changes occurring in natural seawater. The error bars represent standard deviation. Full size image The subsamples collected over time during the incubations were observed using transmission electron microscopy (TEM) and scanning electron microscopy (SEM) with the purpose of investigating the change in morphology and elemental composition of detrital organic matter during cell degradation. The spherical or ellipsoidal shapes of Synechococcus dominated the initial samples ( Fig. 2a,b ). Other phytoplankton species were much less frequently observed compared with the added Synechococcus cells, and were considered unimportant in this experimental setting. Also present were extracellular fibrillar structures, which are similar in morphology to extracellular polymeric substances (EPS) commonly found in marine environments [9] , [10] . Similar structures of EPS have also been widely observed in cyanobacterial cultures [11] . Some EPS were present in initial cell cultures, but they were more abundant than intact cells in degraded samples. After 2 days of incubation in experiments with bacteria present, most cells had lysed and lost their shapes ( Fig. 2c,d ). Lysed cells were surrounded by an abundance of EPS, although much of this EPS was not visibly attached to cells. Newly produced EPS would most likely originate from cyanobacteria or heterotrophic bacteria [12] , [13] , since other organisms were a minor component. TEM pictures of both intact ( Fig. 2c,e ) and thin-sectioned samples ( Fig. 2d,f ) showed that many of the EPS fibrils were progressively rearranged to form dark, sharp and elongated clusters during the incubation from day 2 to day 15. 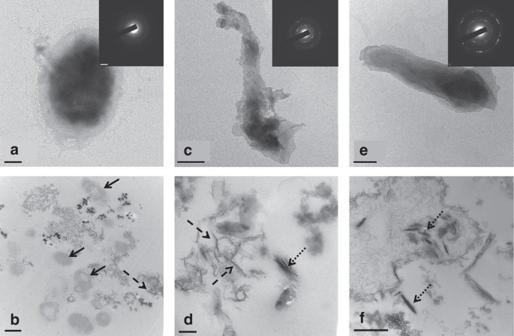Figure 2: TEM images of decomposingSynechococcuscells. Samples were taken during the dark incubation ofSynechococcuscells in coastal seawater with natural microbial communities, initially (t0, (a,b)), after 2 days (t2, (c) and (d)) and after 15 days (t15, (e,f)). Selected area electron diffraction patterns are pictured ina,c, ande, and reflect the crystallographic axis orientation changing across grain boundaries; polycrystalline structures were characterized by rings of luminous points incande.b,dandfare images of 80-nm thick thin sections of samples after chemical fixation.Synechococcuscells were marked by solid arrows inb. Fibrillar-like EPS were marked by dash arrows inbandd. Electronically dense fibrillar-like particles were marked by dot arrows indandf(Scale bars, 200 nm ina, 500 nm inb, 100 nm inc, 100 nm ind, 100 nm ineand 500 nm inf). Figure 2: TEM images of decomposing Synechococcus cells. Samples were taken during the dark incubation of Synechococcus cells in coastal seawater with natural microbial communities, initially (t 0 , ( a , b )), after 2 days (t 2 , (c) and (d)) and after 15 days (t 15 , ( e , f )). Selected area electron diffraction patterns are pictured in a , c , and e , and reflect the crystallographic axis orientation changing across grain boundaries; polycrystalline structures were characterized by rings of luminous points in c and e . b , d and f are images of 80-nm thick thin sections of samples after chemical fixation. Synechococcus cells were marked by solid arrows in b . Fibrillar-like EPS were marked by dash arrows in b and d . Electronically dense fibrillar-like particles were marked by dot arrows in d and f (Scale bars, 200 nm in a , 500 nm in b , 100 nm in c , 100 nm in d , 100 nm in e and 500 nm in f ). Full size image In addition, TEM selected area electron diffraction patterns showed that polycrystalline structures of several hundred nanometers in length formed after 2 days of degradation. These structures were commonly observed in both day 2 and day 15 incubation samples ( Fig. 2c,e ), but were rare in samples incubated in the sterilized medium. The polycrystalline structures were morphologically similar to the silicate mineral smectite that has been found to associate with organic matter in California continental margin sediments [14] . It has been suggested that smectite can be produced authigenically at low temperatures in association with bacteria [15] . Energy dispersive X-ray spectroscopy (EDS) mounted on SEM demonstrated that these atomically-dense structures were enriched in Si and Mg compared with adjacent intact Synechococcus cells ( Fig. 3 ). We did not detect any accumulation of these crystals inside cyanobacterial cells. 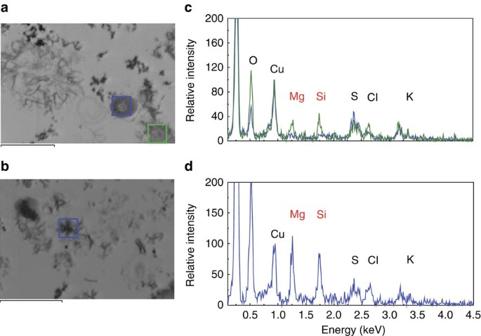Figure 3: Scanning transmission electron microscope images and EDS spectra of decomposingSynechococcuscells. Images were taken on thin-sectioned samples (80 nm) collected during dark incubation ofSynechococcuscells after 2 days (a) and 15 days (b). After 2 days, the EDS spectrum (blue spectrum inc) of an intact cyanobacterial cell (blue box ina) shows the absence of Mg and Si inside the cell. However, the EPS adjacent to the cell (green box ina) accumulated both Mg and Si (Green spectrum inc), as did the EPS in the more degraded samples (blue box inband blue spectrum ind). The observed Cu was from the copper grid holder (Scale bar, 1 μm). Figure 3: Scanning transmission electron microscope images and EDS spectra of decomposing Synechococcus cells. Images were taken on thin-sectioned samples (80 nm) collected during dark incubation of Synechococcus cells after 2 days ( a ) and 15 days ( b ). After 2 days, the EDS spectrum (blue spectrum in c ) of an intact cyanobacterial cell (blue box in a ) shows the absence of Mg and Si inside the cell. However, the EPS adjacent to the cell (green box in a ) accumulated both Mg and Si (Green spectrum in c ), as did the EPS in the more degraded samples (blue box in b and blue spectrum in d ). The observed Cu was from the copper grid holder (Scale bar, 1 μm). Full size image Chemical analysis provides further support for the idea that Si becomes associated with EPS during the degradation of cyanobacteria cells. Biogenic silicate concentration, [BSi], increased to as much as 52±7 μmol l −1 after 7 days of degradation of the two strains ( Fig. 1 ), compared with the much lower [BSi] in cultures incubated in the sterilized medium (average 6.5±4.5 μmol l −1 ) and in seawater without cyanobacteria added (average 2.8±1.8 μmol l −1 ). BSi that formed during degradation decreased in concentration after 7 days, with only 13±3 μmol l −1 remaining on day 30 of the incubation. The ratio Si:C (BSi to particulate organic carbon) was elevated (as high as 0.056) in cultures with degrading cyanobacteria, in contrast to the constant and lower Si:C (0.003) in cells incubated in sterile medium ( Fig. 1 ). Meanwhile, the relative abundance of glycine in dissolved hydrolysable amino acids was significantly enriched at the end of incubation, which supports evidence that Si-associated amino acids are enriched in glycine [16] ( Supplementary Fig. 2 ). All these results observed in experiments with microbes present compared with the sterile control show the importance of the degradation process to Si deposition, whatever the mechanism. The subsequent decrease in BSi after 2 weeks is probably owing to both dissolution of BSi and loss of organic matter, whether from cyanobacteria or from EPS [17] . The Si:C of ~0.03 to 0.06 in our Synechococcus degradation experiments are lower than ratios found in diatoms (~0.13) [18] . But given the higher abundance of picophytoplankton biomass in the open ocean [2] , cyanobacterial degradation and subsequent formation of Si-organic matter (Si-OM) association (that might serve as an important source of ballast) could account for up to 50% of the BSi inventory in the surface water ( Supplementary Table 1 ). We considered possible mechanisms for Si deposition in our experiments. First, cyanobacteria-derived EPS-associated Si and Mg do not result from silicate scavenging by brucite, [Mg(OH) 2 ], a mineral that forms in seawater when pH increases as a result of photosynthesis [19] . No brucite crystals were observed in cyanobacteria cultures (pH=8.9) incubated in coastal seawater, nor in cultures incubated in sterile seawater. Although CO 2 is formed when cyanobacteria degrade over time, the pH during our incubations ranged between 7.5 and 8.1, which is not favorable for brucite formation (pH>10) [19] . Second, EPS-associated Si does not originate from silicic acid dissolved from diatoms present in the coastal seawater used in the incubations, because very few diatoms were present, and silicic acid concentrations in all incubations, from 30 to 99 μmol l −1 ( Supplementary Fig. 1 ), were much lower than opal solubility of 1,600 μmol l −1 (ref. 20 ), but similar to silicic acid levels in most coastal environments as well as deep water of the North Atlantic Ocean ( Supplementary Fig. 3 ). A third more likely explanation for the presence of EPS-associated Si and Mg is that EPS incorporates the Si from the Synechococcus cells [21] . Recent studies of both field and culture samples demonstrate that living cyanobacteria cells can accumulate significant amounts of Si [22] . As these cells begin to degrade, cell lysis could cause a local elevation of silicic acid concentration near the cells. Cell lysis can also produce large amounts of EPS, which could provide an organic template that selectively incorporates the elevated Si. The progressive accumulation of Mg and Si in EPS may be related to the formation of the nano- to micro-crystalline particles we observed during degradation of the Synechococcus . In previous studies, fine grained silicate was also observed in fresh water biofilm and bacterial cultures [15] . Marine particles from Bermuda rise Mg–Si deposition was not limited to laboratory samples. To study the existence of EPS-Si in natural particles, samples were collected at a site northeast of Bermuda in October 2011, as part of the BARFlux project. This site on the Bermuda rise has limited terrestrial input. Suspended particles of 0.8–5 μm in size collected from a variety of depths were made up of three major types of particles, organic matter-rich particles here called ‘micro-blebs’ ( Fig. 4a , Supplementary Fig. 4 ) ( c.f. , [14] ), carbonaceous coccolith-like fragments ( Fig. 4a ) and siliceous diatom-like frustules ( Fig. 4b ). The coccolith and diatom frustules had distinguishable geometrical structures, while micro-blebs had no well-defined or regularly arranged structures, but appeared to be loosely aggregated organic materials. These micro-blebs were also different from diatom frustules and coccoliths in their elemental compositions. EDS analysis suggested that micro-blebs were characterized by elevated Si and Mg, which is similar to the EPS-associated Si observed in degrading cyanobacteria ( Fig. 4 , Supplementary Table 2 ). Diatom frustules were specifically enriched in Si but not Mg, and coccoliths had a high abundance of Ca and Mg but not Si. Besides being enriched in Si and Mg, neither micro-blebs nor the EPS-Si surrounding degrading cyanobacteria had regularly arranged biogenic geometrical structures. BSi analysis on parallel filters suggests that particles in the size range 0.8–5 μm accounted for the majority of BSi ( Supplementary Fig. 3 ). These visual, chemical and physical similarities lead us to speculate that EPS-Si produced during the degradation of marine cyanobacteria is one of the possible origins of the micro-blebs observed in marine particles. The Al seen in the spectra of marine particles was likely from the aluminium sample holder used in SEM as Al was absent in samples where the aluminium holder was not used ( Supplementary Fig. 5 ). Therefore, dust particles, which are usually enriched in Al and Si, probably have a limited contribution to these micro-blebs. Fecal pellets were found only in particles larger than 5 μm, so may not be a major source of these elements, but potentially function in packaging small particles in surface water and releasing these particles in mesopelagic water during decomposition [23] . 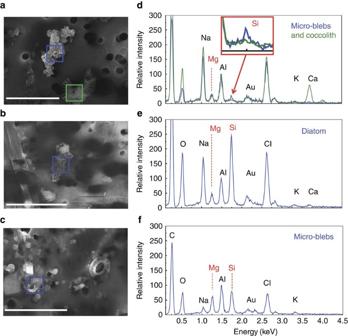Figure 4: SEM images of particles from Bermuda Rise. SEM images (a–c) and EDS spectra (d–f) of marine suspended particles collected from 2,000-m water depth (a,b,dande) and from 50 m (c,f) near the Bermuda Rise. A micro-bleb (blue box inaand blue spectrum ind) and a coccolith fragment (green box inaand green spectrum ind) are shown inaandd, and a fragment of diatom frustule is shown as blue box inband blue spectrum ine. A higher loading of particles is observed in surface water (c). The elemental compositions of micro-blebs were scanned by EDS. Micro-blebs from both surface (blue spectrum inf) and 2,000 m (blue spectrum ind) were enriched in both Mg and Si. Enrichment of Al is from the aluminium holder (Scale bars, 5 μm ina, 9 μm inband 7 μm inc). Figure 4: SEM images of particles from Bermuda Rise. SEM images ( a – c ) and EDS spectra ( d – f ) of marine suspended particles collected from 2,000-m water depth ( a , b , d and e ) and from 50 m ( c , f ) near the Bermuda Rise. A micro-bleb (blue box in a and blue spectrum in d ) and a coccolith fragment (green box in a and green spectrum in d ) are shown in a and d , and a fragment of diatom frustule is shown as blue box in b and blue spectrum in e . A higher loading of particles is observed in surface water ( c ). The elemental compositions of micro-blebs were scanned by EDS. Micro-blebs from both surface (blue spectrum in f ) and 2,000 m (blue spectrum in d ) were enriched in both Mg and Si. Enrichment of Al is from the aluminium holder (Scale bars, 5 μm in a , 9 μm in b and 7 μm in c ). Full size image Contribution of cyanobacterial BSi to Si and C cycling The potential contribution of Synechococcus -derived BSi to silicon and carbon flux was calculated for the Bermuda Rise site using estimates of various parameters from North Atlantic Ocean data ( Supplementary Table 1 and references therein). The percentage of Si-associated OM in BSi was calculated from the EDS spectra as the ratio of Si concentrations in the Si-OM particles (six particles, as in Supplementary Table 2 ) to the total Si concentrations in all the particles collected at 2,000-m depth (21 particles, as in Supplementary Table 2 ), or 11%. Si concentrations mentioned here are the normalized Si concentrations that were relative to Al, because Al is an artifact of the Al sample holder. This eliminates the effect from scanning time of each SEM spectra. Thus we assumed that 11% of exported BSi is in the form of Si-OM, of which the Si:C ratio of 0.042 (average Si:C ratios from the later stage of incubations) was assumed for these Si-OM particles. This results in a Si-OM-derived POC flux of 0.011 g C m −2 per day, which is around 43% of the POC flux leaving the euphotic zone (0.03 g C m −2 per day) [2] . Synechococcus Si export can also be estimated from Synechococcus carbon export and the Si:C ratio, where Synechococcus carbon export was estimated from POC export, 0.026 g C m −2 per day, and the contribution of Synechococcus to POC flux, 2–13% ( Supplementary Table 1 and references therein). This results in a Synechococcus Si export of 2–12 μmol Si m −2 per day out of the euphotic zone, and accounts for 0.5–3% of the total annual Si export. This estimate of the contribution of Synechococcus to Si export is in the range of our calculation above that 11% of the Si in the deep ocean is in the form of Si-OM. This supports our suggestion that Si-OM in the deep ocean on the Bermuda rise may originate from Synechococcus -derived Si. In the surface water near Bermuda, Synechococcus -derived BSi (Syn-BSi) standing stock was estimated by multiplying Synechococcus biomass by the Syn-BSi production coefficient [24] . This production coefficient was calculated by dividing the average BSi produced by the fresh cell biomass added to the incubation, which indicates the BSi production of Synechococcus under ideal conditions. Syn-BSi standing stock accounts for 50% of the BSi inventory in the surface water, thus implying that half of the BSi in the surface water may originate from Synechococcus . The following uncertainties should be considered with regard to the Syn-BSi budget in the open ocean: (1) The relative abundance of Si-OM in total BSi was calculated from EDS data, which scans only the surface of particles; thus the concentration reflects the elemental composition at the particle surface instead of the entire particle. It is possible that this method overestimates Si concentrations in the Si-OM particles since Si and Mg may preferentially deposit on the surface of organic matter. (2) The Si:C ratio used in the calculations was from a 30-day Synechococcus incubation where cells were degraded solely by heterotrophic bacteria. It is not clear how Si:C would change over a much longer time scale, and also how other processes like zooplankton grazing change the Si:C ratio. Further work should be conducted to better evaluate these uncertainties. Cyanobacterial silicification has been observed previously in microfossils and in modern extreme environments like hot springs and sediments where amorphous silicate is supersaturated and pH is often extreme [25] , [26] , [27] , [28] . However, the EPS-silicate found in this study is different, as it is deposited in the open ocean with its mild pH and opal undersaturation. Previous studies demonstrate that more than half of the biogenic silicate in the open ocean is detrital, and is not derived from siliceous phytoplankton like diatom as was previously thought [29] . Our finding of Mg–Si deposits originating during decomposition of cyanobacteria implies a new source of detrital silicate to the oceans in addition to siliceous phytoplankton. The close association between Si and EPS could also provide protection from remineralization for the EPS, while the increased Si content could contribute to density-driven particle export [4] . The EPS structure might also slow chemical dissolution of silica in the euphotic zone as suggested by the relatively constant Si:C ratio at the end of the Synechococcus incubation. If we assume that the Si:C ratio observed in the incubation is applicable in the deep ocean, Si-enriched organic matter could account for as much as 43% of the export production at Bermuda. Therefore, it must be considered in studies of particle flux in the open ocean. This finding provides an additional explanation for recent findings that pico- and nano-phytoplankton can be exported into the deep ocean [6] , [7] , [8] . Further investigation is needed to elucidate the contribution of this new type of biogenic silicate to the particle flux in marine environments. Culture preparation Strains of the cyanobacteria Synechococcus sp. CCMP2370 and CCMP1334 (Bigelow Laboratory) were grown in sterile L1 medium prepared with 0.2-μm filtered coastal seawater (Stony Brook Harbor). The cultures were incubated at 20 °C with a 16:8 illumination cycle of ~1 × 10 4 μmol quanta m −2 sec −1 . Cells were harvested at the end of the exponential growth stage or early stationary stage by centrifugation at 5,250 g for 40 min. Pellets of cells were rinsed with and resuspended in 0.2 μm filtered coastal seawater. Chlorophyll a concentrations in collected cultures were estimated from the whole cell spectra from 600 nm to 800 nm using a Perkin Elmer UV-VIS spectrophotometer [30] . We measured chlorophyll a as a way of ensuring that we were adding the same amount of cells to each incubation. Incubation of cyanobacterial cells Harvested cyanobacterial cells were added to coastal seawater (Stony Brook Harbor) that was filtered through 178-μm mesh to remove large zooplankton. Cultures were adjusted to have the same chlorophyll concentrations. The incubations were conducted in sterilized polycarbonate flasks in the dark at 22–24 °C. Subsamples were collected after 0, 2, 7, 15 and 30 days. After centrifugation at 5,250 g for 40 min, both the supernatants and pellets were collected as surrounding water and particle samples, respectively. No increase of plankton larger than 1 μm was observed in 30-day incubations. Incubations of coastal seawater without Synechococcus present were also carried out under identical conditions as a blank control. A parallel incubation of Synechococcus CCMP2370 added to autoclaved coastal seawater was used as a sterile control. pH was measured in each subsample using a Ross electrode. Marine suspended particle collection Marine suspended particles were collected from a site northeast of Bermuda (33.68°N, 57.6°W) on the R/V Endeavour in October 2011 (BaRFlux I). About 8 l of seawater was collected from various depths using Niskin bottles on a rosette and transferred to a 10-l acid rinsed container, which was then filtered through in-line polycarbonate filter holders with 5 μm and 0.8 μm polycarbonate filters in sequence. The filtrate was further filtered through 0.2-μm polycarbonate filters using a Nalgene polysulfone filtration system. Glassware was avoided during sampling and storage. All filters were frozen until analysis of BSi and electron microscopy. Bulk chemical analysis BSi was collected during Synechococcus incubations on 0.2-μm polycarbonate filters. The incubation samples as well as Bermuda samples were extracted with 0.2 M NaOH and measured colorimetrically as [H 4 SiO 4 ] in the extract [31] . Silicic acid (H 4 SiO 4 ) concentrations in 0.2 μm filtered seawater samples were analyzed using the molybdate blue spectrophotometric method [32] on a Lachat flow injection colorimeter. POC samples from both Synechococcus incubations and Bermuda Rise seawater was collected by filtering through combusted 0.7 μm Glass Fiber Filters (Whatman). Filters were desiccated at 50 °C after removing carbonate with HCl vapor. POC and particulate nitrogen on filters were analyzed on Thermo NC analyzer. Electron microscopy One-ml subsamples were taken from incubations and centrifuged at 4,000 g for 20 min. The pellets were washed and resuspended in 0.1 ml of distilled water. One drop of the sample was fixed onto 300-mesh carbon-coated copper grids for 60 s before being air-dried for TEM analysis. Prepared grids were viewed on a JEOL JEM-1400 TEM at an accelerating voltage of 120 kV. Selected area diffraction mode was applied on interesting parts of the samples. Thin sections were prepared by centrifuging 45-ml subsamples from cyanobacterial incubations at 5,525 g for 40 min. The pellets were fixed with 3% glutaraldehyde/0.05 M phosphate buffer (pH=7), and kept at 4 °C overnight. The samples were then dehydrated with ethyl alcohol. The samples were then stained with lead citrate and uranyl acetate. After being embedded in Epon resin, the samples were cut into ultrathin 80-nm sections with a Reichert-Jung Ultracut E Ultramicrotome. Thin sections were placed on Formvar-coated slot copper grids, and TEM images were taken using an FEI BioTwinG2 Transmission Electron Microscope. The same grid was further analyzed on a JEOL 7600 analytical SEM with an Oxford energy dispersive X-ray spectrometer in STEM mode. Filtered particles from the Bermuda Rise sampling site were dried at 55 °C overnight. The dried filters were coated with gold on an aluminium sample holder, and SEM images were taken using a JEOL 7600 analytical SEM with an Oxford energy dispersive X-ray spectrometer . Amino acid analysis Dissolved hydrolysable amino acids and particulate amino acids were analyzed during the degradation experiment. Individual amino acids were measured after hydrolysis in both particles (pellets that contained cell detritus and other particles) and surrounding seawater (supernatant) from the Synechococcus incubations [33] . Samples were hydrolyzed at 110 °C in 6 N HCl (Trace metal basis, Sigma-Aldrich) and 0.11 μmol l −1 ascorbic acid (Sigma-Aldrich) for 20 h. The acid was removed by nitrogen sparging. D - and L -amino acids were chirally derivatized with o-phthaldialdehyde (Sigma-Aldrich) and N-isobutyryl- L -cysteine (Fluka). D - and L - amino acids were separated by high performance liquid chromatography with fluorescence detection (Excitation/Emission=330/445 nm). Only L -amino acids were included in calculations of dissolved and particulate amino acid composition. Pierce H amino acid standard was mixed with individual D -amino acid standards to result in a mixed standard for both D - and L -amino acids; beta-alanine and gamma-aminobutyric acid were also added. How to cite this article: Tang, T. et al . Silicate deposition during decomposition of cyanobacteria may promote export of picophytoplankton to the deep ocean. Nat. Commun. 5:4143 doi: 10.1038/ncomms5143 (2014).